BRCA1 haploinsufficiency for replication stress suppression in primary cells BRCA1 —a breast and ovarian cancer suppressor gene—promotes genome integrity. To study the functionality of BRCA1 in the heterozygous state, we established a collection of primary human BRCA1 +/+ and BRCA1 mut/+ mammary epithelial cells and fibroblasts. Here we report that all BRCA1 mut/+ cells exhibited multiple normal BRCA1 functions, including the support of homologous recombination- type double-strand break repair (HR-DSBR), checkpoint functions, centrosome number control, spindle pole formation, Slug expression and satellite RNA suppression. In contrast, the same cells were defective in stalled replication fork repair and/or suppression of fork collapse, that is, replication stress. These defects were rescued by reconstituting BRCA1 mut/+ cells with wt BRCA1. In addition, we observed ‘conditional’ haploinsufficiency for HR-DSBR in BRCA1 mut/+ cells in the face of replication stress. Given the importance of replication stress in epithelial cancer development and of an HR defect in breast cancer pathogenesis, both defects are candidate contributors to tumorigenesis in BRCA1-deficient mammary tissue. Germ line BRCA1 mutations increase greatly the risk of breast and ovarian cancer [1] , [2] , [3] . While all cells of males and females with germline BRCA1 mutations exhibit a heterozygous BRCA1 mut/+ genotype, cancer develops primarily in females, often at young ages and almost exclusively affects the breast and ovaries. Why BRCA1 is largely a breast and ovarian cancer susceptibility gene, why males are largely protected from BRCA1 cancer and how an ostensibly normal mammary epithelial cell in a BRCA1 mutation carrier ( BRCA1 mut/+ ) gives rise to breast cancer cells are largely unknown. In addition, there is insufficient mechanistic insight into BRCA1 breast tumorigenesis on which to base rational preventive strategies. Their design will, in part, require a deeper appreciation of the biological properties of a heterozygous but ostensibly normal, mammary epithelium ( BRCA1 mut/+ ). The tumour-suppressing BRCA1 protein is an E3 ubiquitin ligase and a multi-functional scaffold that binds numerous partner proteins [4] , [5] . It plays a key role in genome integrity maintenance, which appears to be an essential component of its tumour-suppressing function [2] , [5] , [6] . A BRCA1 loss of heterozygosity (LOH) event is a consistent characteristic of fully developed BRCA1 -linked tumour cells. Two generic models describe the chain of events that precede it and the concomitant emergence of mammary tumour cells (human mammary epithelial cells (HMECs)). In one, HMECs, despite being heterozygous, are histologically and biologically normal before the emergence of LOH. They fail to exhibit a significant defect in BRCA1 function. Here key events that transform a cell to malignancy follow the loss of all BRCA1 functions at the LOH event and are often preceded by acquisition of a p53 mutation that sustains cell viability in the face of emerging genome disorder [7] . In the other model, BRCA1 mut/+ HMECs are haploinsufficient for the performance of one or more BRCA1 functions even before any signs of a neoplastic cell phenotype emerge. This model implies that, from the time that mammary epithelial development is complete or at some relatively early time thereafter, BRCA1 mut/+ HMECs cannot perform all BRCA1 genome integrity maintenance functions at normal amplitude. These abnormalities may increase the likelihood that steps in the mammary tumorigenesis process begin long before they become clinically apparent. In this regard, there is growing evidence of a defect in normal mammary epithelial progenitor differentiation in histologically normal, BRCA1 heterozygous mammary tissue [8] , [9] , [10] , [11] , implying that the second model is more likely valid than the first. Thus, determining whether BRCA1 heterozygosity confers haploinsufficiency on HMECs for any of the multiple, known, BRCA1 functions is a potentially valuable step in achieving a better understanding of BRCA1 mutation-driven cancer predisposition. In this regard, we have analysed a new collection of primary mammary BRCA1 mut/+ epithelial cells and skin fibroblasts obtained from BRCA1 mutation carriers for such functions. Primary cell genotyping and lineage determination Established elements of BRCA1 function were analysed in freshly isolated, morphologically non-neoplastic, primary HMECs and skin fibroblasts derived from multiple BRCA1 +/+ and BRCA1 mut/+ tumour-free women. 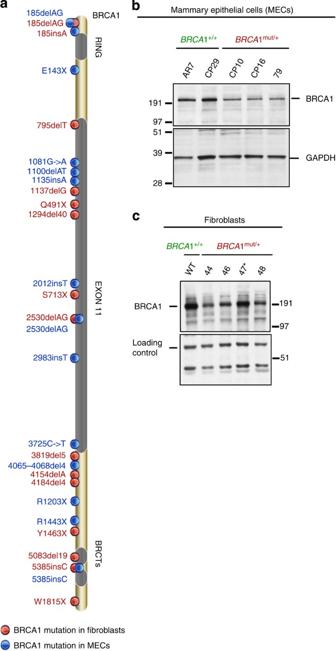Figure 1: Distribution ofBRCA1mutations and BRCA1 protein in cells derived fromBRCA1mutation carriers. (a) Cells were derived from skin punch biopsies and prophylactic mastectomies performed onBRCA1mutation carrying women. (b) Western blot analysis of total BRCA1 protein levels inBRCA1mut/+andBRCA1+/+HMEC lines. Equivalent amounts of whole-cell lysate (prepared in NETN300) were electrophoresed, blotted and the blots probed with an anti-BRCA1 monoclonal Ab (SD118). GAPDH served as a loading control. (c) Western blot analysis of BRCA1 protein levels in the nuclear fraction ofBRCA1mut/+andBRCA1+/+fibroblast strains. Cells were pre-lysed in pre-extraction buffer (PEB, details in Materials and Methods), and the pellet was re-suspended in NETN400 buffer to prepare a nuclear extract. The intense BRCA1 band in 47 (185delAG, marked by an asterisk) is likely the previously discovered truncated product of this mutant allele45. A non- specific band served as the loading control. Twenty-three primary BRCA1 mut/+ fibroblast cultures were derived from skin punch biopsies, and 15 primary BRCA1 mut/+ HMEC cultures were generated from individual prophylactic mastectomy samples ( Table 1 ). HMECs were cultured in serum-free medium. Table 1 Primary fibroblast and HMEC strains ( BRCA1 +/+ and BRCA1 mut/+ ) used in this study. Full size table The properties of BRCA1 mut/+ HMECs were compared with BRCA1 +/+ HMECs ( N =7), freshly derived from reduction mammoplasty tissue, and those of BRCA1 mut/+ skin fibroblasts with freshly isolated BRCA1 +/+ fibroblasts ( N =11; Table 1 ). Mutations in BRCA1 mutant fibroblasts and HMECs were confirmed by homogenous Mass-Extend (hME) analysis [12] and by direct BRCA1 gene sequencing ( Supplementary Fig. 1a–c ). Together, this collection of BRCA1 mut/+ mutations spans nearly the entire BRCA1 genome ( Fig. 1a ). Figure 1: Distribution of BRCA1 mutations and BRCA1 protein in cells derived from BRCA1 mutation carriers. ( a ) Cells were derived from skin punch biopsies and prophylactic mastectomies performed on BRCA1 mutation carrying women. ( b ) Western blot analysis of total BRCA1 protein levels in BRCA1 mut/+ and BRCA1 +/+ HMEC lines. Equivalent amounts of whole-cell lysate (prepared in NETN300) were electrophoresed, blotted and the blots probed with an anti-BRCA1 monoclonal Ab (SD118). GAPDH served as a loading control. ( c ) Western blot analysis of BRCA1 protein levels in the nuclear fraction of BRCA1 mut/+ and BRCA1 +/+ fibroblast strains. Cells were pre-lysed in pre-extraction buffer (PEB, details in Materials and Methods), and the pellet was re-suspended in NETN400 buffer to prepare a nuclear extract. The intense BRCA1 band in 47 (185delAG, marked by an asterisk) is likely the previously discovered truncated product of this mutant allele [45] . A non- specific band served as the loading control. Full size image To determine the lineage of cells that grew out of our primary tissue samples under the culturing conditions used, we carried out flow cytometry (FACS)-based analysis of lineage markers (CD44, CD49f, CD24 and EpCAM). In this study, our primary BRCA1 mut/+ and BRCA1 +/+ HMEC cultures were similarly enriched in early basal (CD44 high , CD24 low , CD49f high EpCAM low ) relative to luminal progenitor cells (CD44 low , CD49f low , CD24 high , EpCAM high ) [9] , [13] ( Supplementary Fig. 2a ). For this analysis, MCF7 was used as a luminal cell line control and MCFDCIS.com as a basal cell line control. Furthermore, western blot analysis of whole-cell (for HMECs) and nuclear extracts (for fibroblasts) revealed that full-length BRCA1 expression in BRCA1 mut/+ HMEC ( Fig. 1b and Supplementary Fig. 2c ) and fibroblast strains ( Fig. 1c and supplementary Fig. 2b ) was lower than that detected in wt BRCA1 +/+ lines. This was in keeping with the proven genetic heterozygosity in these cells. As BRCA1 is much more abundant in S and G2 than in G1, we only analysed wt and heterozygous HMEC and fibroblast cultures that exhibited similar cell cycle profiles and BUdR uptake (see for example, Supplementary Fig. 2c ). Non-DNA repair-driven BRCA1 genome integrity functions BRCA1 exhibits two types of genome integrity maintenance functions—those that are directed towards the repair of DNA damage and checkpoint control, and others that sustain genome integrity by contributing to homeostatic functions that are not necessarily driven by DNA damage. In this context, we asked whether the lower expression of BRCA1 in BRCA1 mut/+ cell cultures was associated with a deficiency in the latter BRCA1 functions. BRCA1 is required for the maintenance of centrosome number [14] , mitotic spindle pole formation [15] , [16] , [17] , mammary development through the regulation of master genes like Slug [11] and heterochromatin-based satellite RNA suppression [18] . Each of these functions was compared in heterozygous ( BRCA1 mut/+ ) and control ( BRCA1 +/+ ) cells. Spindle formation was analysed by staining mitotic cells with a TPX2 antibody. No abnormal spindle formation was detected in BRCA1 mut/+ cells ( Fig. 2a and Table 1 ). The effects of robust BRCA1 depletion on this function have been documented [15] . 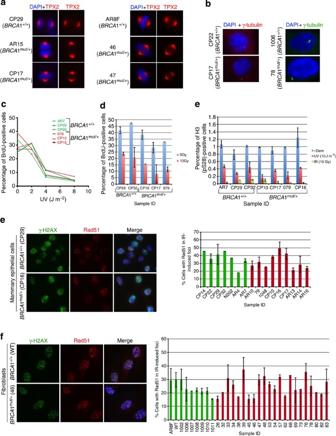Figure 2: Spindle pole formation, centrosome number, checkpoint activation and Rad51 recruitment to DSB. (a) Representative images of HMECs (left panel) and skin fibroblasts (right panel), fromBRCA1mut/+andBRCA1+/+were immunostained with an anti- TPX2 Ab to detect spindles;n=50 spindles were analysed for each strain. A summary of all strains that were tested in this assay is listed insupplementary Table 1. (b) Centrosome number was determined by immunostaining HMECs (left panel) and fibroblasts (right panel) with Ab to γ-tubulin;n=50 cells for each line were counted and cells with centrosomes ≤2 were considered normal. A summary of the lines that were tested is presented inSupplementary Table 1. (c) S-phase checkpoint in response to UV- and IR-induced DNA damage in control andBRCA1mut/+strains. ThreeBRCA1+/+(AR7, CP22 and CP29) and threeBRCA1mut/+HMEC strains (79, CP10 and CP16) were irradiated with increasing doses of UV (left panel). For IR-induced S-phase checkpoint analysis (right panel), cells were exposed to IR (10 Gy, red). Non-irradiated cells (0 Gy, blue) served as controls. Error bars indicate the s.d. between the results of three, independent experiments. (d) G2/M checkpoint activation in response to UV- and IR- induced DNA damage inBRCA1mut/+and control cells.BRCA1+/+andBRCA1mut/+cells were irradiated with either UV (10 J m−2) or IR (10 Gy), allowed to recover for 2 h and then harvested for FACS analysis. The percentage of cells in mitosis was determined by staining cells with propidium iodine (PI) and phosphorylated histone H3 (S28) antibody. Mock-irradiated (-Dam) cells served as controls. (e) HMECs and (f) fibroblasts were exposed to IR (10 Gy) and allowed to recover for 4 h. Cells were fixed and co-immunostained with Abs to γ-H2AX and Rad51. Graphs depicting the fraction of cells with Rad51 foci that co-localized with γ-H2AX foci for each line are plotted for both HMECs and fibroblasts (right panels ineandf). Mean and s.d. of at least three experiments for each strain are shown. wtBRCA1+/+(green) andBRCA1mut/+(red) lines. Figure 2: Spindle pole formation, centrosome number, checkpoint activation and Rad51 recruitment to DSB. ( a ) Representative images of HMECs (left panel) and skin fibroblasts (right panel), from BRCA1 mut/+ and BRCA1 +/+ were immunostained with an anti- TPX2 Ab to detect spindles; n =50 spindles were analysed for each strain. A summary of all strains that were tested in this assay is listed in supplementary Table 1 . ( b ) Centrosome number was determined by immunostaining HMECs (left panel) and fibroblasts (right panel) with Ab to γ-tubulin; n =50 cells for each line were counted and cells with centrosomes ≤2 were considered normal. A summary of the lines that were tested is presented in Supplementary Table 1 . ( c ) S-phase checkpoint in response to UV- and IR-induced DNA damage in control and BRCA1 mut/+ strains. Three BRCA1 +/+ (AR7, CP22 and CP29) and three BRCA1 mut/+ HMEC strains (79, CP10 and CP16) were irradiated with increasing doses of UV (left panel). For IR-induced S-phase checkpoint analysis (right panel), cells were exposed to IR (10 Gy, red). Non-irradiated cells (0 Gy, blue) served as controls. Error bars indicate the s.d. between the results of three, independent experiments. ( d ) G2/M checkpoint activation in response to UV- and IR- induced DNA damage in BRCA1 mut/+ and control cells. BRCA1 +/+ and BRCA1 mut/+ cells were irradiated with either UV (10 J m −2 ) or IR (10 Gy), allowed to recover for 2 h and then harvested for FACS analysis. The percentage of cells in mitosis was determined by staining cells with propidium iodine (PI) and phosphorylated histone H3 (S28) antibody. Mock-irradiated (-Dam) cells served as controls. ( e ) HMECs and ( f ) fibroblasts were exposed to IR (10 Gy) and allowed to recover for 4 h. Cells were fixed and co-immunostained with Abs to γ-H2AX and Rad51. Graphs depicting the fraction of cells with Rad51 foci that co-localized with γ-H2AX foci for each line are plotted for both HMECs and fibroblasts (right panels in e and f ). Mean and s.d. of at least three experiments for each strain are shown. wt BRCA1 +/+ (green) and BRCA1 mut/+ (red) lines. Full size image Similarly, we found that none of the BRCA1 mut/+ and BRCA1 +/+ cells contained greater than 2 centrosomes, implying that centrosome maintenance was normal in these different BRCA1 mut/+ strains ( Fig. 2b and Supplementary Table 1 ). Although we did not detect any evidence of centrosome amplification in multiple BRCA1 heterozygous cells, other work [7] with BRCA1 heterozygous tissue has detected a small increase of centrosome amplification (~5%) in the epithelial cells of heterozygous mammary tissue compared with 2.5% in wt tissue. De-repression of satellite RNA transcription is also a feature of BRCA1 mutant tumours [18] . Furthermore, Brca1 heterozygous cells do not show evidence of satellite de-repression [18] . To test whether this phenotype was present in heterozygous BRCA1 HMECs, two approaches were employed. Quantitative RT-PCR (q-RT-PCR) was performed for alpha satellite variants (SATIII, SATa and mcBox). Satellite RNA transcript levels were also estimated by RNA FISH directed at another satellite RNA, HSATII. Very low levels of satellite RNA were present in primary HMECs, making it difficult to detect any satellite RNA signal by these methods ( Supplementary Fig. 3a and b ). To address the effect of BRCA1 heterozygosity on Slug expression [11] , we compared the Slug level in BRCA1 +/+ and BRCA1 mut/+ HMECs by western blot analysis. In these experiments, MCF7 (a luminal breast cancer line) was used as a negative control and MDA-MB-231 (a basal line) was used as a positive control. No reproducible difference in Slug expression was detected between the BRCA1 +/+ and BRCA1 mut/+ strains that were tested ( Supplementary Fig. 3c ). Addition of serum [11] had similar effect on Slug expression in BRCA1 +/+ and BRCA1 mut/+ strains. DNA damage checkpoints BRCA1 plays an important role in regulating both the S phase and G2 checkpoints after DNA damage [19] , [20] . The efficiency of post-damage checkpoint activation was also tested in BRCA1 heterozygous cells. We failed to detect any significant difference in the ability of BRCA1 +/+ and mut/+ lines to mount either an S phase ( Fig. 2c , left and right panel) or a G2 checkpoint response ( Fig. 2d ) following IR or UV-induced DNA damage. BRCA1 DNA repair functions double-strand break repair BRCA1 plays an essential role in homologous recombination-type double-strand break repair (HR-DSBR) [21] , [22] . Defective HR-DSBR is a well-known property of BRCA1 and related, inherited breast cancers; molecular epidemiology results suggest that it is a risk factor for these cancers [23] , [24] , [25] . BRCA1 is attracted to discrete sites of DSB-containing damage, where it directs a complex HR repair response [5] , [26] . Long-standing results show that in BRCA1 +/− ES cells [27] , HR function is normal until both copies of BRCA1 are inactivated ( BRCA1 −/− ). By contrast, others have reported that targeting one copy of BRCA1 with a mutation (for example, 185delAG) in an established, spontaneously immortal line of human HMECs resulted in a subtle HR defect [28] . Thus, a detailed analysis of multiple, primary human BRCA1 mut/+ and BRCA1 +/+ HMECs and fibroblasts was undertaken to search for evidence of BRCA1 haploinsufficiency for HR-DSBR in this setting. Two, well-validated assays were set up to measure HR-DSBR, by testing the recruitment of Rad51 (an indicator of a key step in HR) [29] to sites of DSBs and by measuring the sensitivity to PARP inhibitors (PI). The first assay clearly showed that BRCA1 mut/+ cells were competent in recruiting Rad51 to sites of DSBs ( Figs 2e,f ). Moreover, like HR-DSBR-competent cells, they were also insensitive to olaparib (a PI). This assay, described below, relies on the observation that sensitivity to a PI is dependent on the existence of an HR defect [30] . Indeed, BRCA1 tumour lines (which lack functional BRCA1 and reveal a defect in HR) are more sensitive to these agents than BRCA1 +/+ cells [31] , [32] . To study the effect of PARP inhibitors in our collection of BRCA1 mut/+ and BRCA1 +/+ cells, a FACS-based cell survival assay of co-cultured cells was employed. Cells were ‘colour-coded’ and tested in pairs, where one cell strain emitted a fluorescent signal (for example, strain A, GFP+) and the other (strain B) did not. Strains A and B were mixed, co-plated and then exposed to a DNA damaging agent of choice. After 7 days of recovery, they were harvested and the relative abundance of each cell population was analysed by FACS ( Fig. 3a ). The ratio of green/non-green or non-green/green cells reflected the relative survival of the two strains. 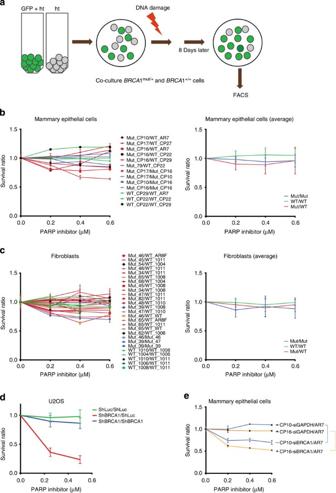Figure 3: FACS-based cell survival assay shows that HR-DSBR is not defective inBRCA1mut/+cells. (a) FACS-based cell survival assay was used to determine the sensitivity of cells to various DNA damage inducing agents.BRCA1mut/+andBRCA1+/+‘colour-coded’ cells were co-plated and exposed to DNA damaging agents. Cell survival data are plotted as a ratio of GFP positive to GFP negative cells. Ratio between WT/WT(Green), Mutant/Mutant (Blue) and Mutant/WT (Red) is plotted in the graphs below. (b) Combinations ofBRCA1mut/+andBRCA1+/+HMECs were exposed to different concentrations of a PARP inhibitor, and the ratio of each of these combinations was plotted (left). The average ratio of WT/WT, Mut/Mut and Mut/WT was also calculated and plotted (right). (c) (Left) Combinations ofBRCA1mut/+andBRCA1+/+fibroblasts were exposed to different concentrations of a PARP inhibitor, and the survival ratio of each of these combinations was plotted (left). An average ratio of WT/WT, Mut/Mut and Mut/WT was also calculated and plotted (right). (d) U20S cells (containing or lacking a GFP reporter) were infected with ShLuc (control) or ShBRCA1 coding lentiviral vectors. Green=ratio of number of ShLuc-treated cells to ShLuc-treated cells, that is (ShLuc/ShLuc), Blue=ratio of number of ShBRCA1-treated cells to ShBRCA1 treated-cells, that is, ShBRCA1/ShBRCA1 and Red=ratio of number of ShBRCA1-treated cells to ShLuc-treated cells, that is, ShBRCA1/ShLuc. Averages of the results of individual experiments are plotted. (e)BRCA1mut/+(CP10 and CP16) were transduced with shRNA directed at GAPDH (siGAPDH) or BRCA1 (siBRCA1). Three days post transfection, combinations of siGAPDH or siBRCA1-transducedBRCA1mut/+HMECs (CP10 and CP16) were co-plated with AR7 (aBRCA1+/+HMEC) and exposed to various doses of a PARP inhibitor. Averages of the results generated by these combinations were plotted. Error bars were calculated as the standard error propagation (SEP) in the ratios of each of the combinations in three independent experiments. Figure 3: FACS-based cell survival assay shows that HR-DSBR is not defective in BRCA1 mut/+ cells. ( a ) FACS-based cell survival assay was used to determine the sensitivity of cells to various DNA damage inducing agents. BRCA1 mut/+ and BRCA1 +/+ ‘colour-coded’ cells were co-plated and exposed to DNA damaging agents. Cell survival data are plotted as a ratio of GFP positive to GFP negative cells. Ratio between WT/WT(Green), Mutant/Mutant (Blue) and Mutant/WT (Red) is plotted in the graphs below. ( b ) Combinations of BRCA1 mut/+ and BRCA1 +/+ HMECs were exposed to different concentrations of a PARP inhibitor, and the ratio of each of these combinations was plotted (left). The average ratio of WT/WT, Mut/Mut and Mut/WT was also calculated and plotted (right). ( c ) (Left) Combinations of BRCA1 mut/+ and BRCA1 +/+ fibroblasts were exposed to different concentrations of a PARP inhibitor, and the survival ratio of each of these combinations was plotted (left). An average ratio of WT/WT, Mut/Mut and Mut/WT was also calculated and plotted (right). ( d ) U20S cells (containing or lacking a GFP reporter) were infected with ShLuc (control) or ShBRCA1 coding lentiviral vectors. Green=ratio of number of ShLuc-treated cells to ShLuc-treated cells, that is (ShLuc/ShLuc), Blue=ratio of number of ShBRCA1-treated cells to ShBRCA1 treated-cells, that is, ShBRCA1/ShBRCA1 and Red=ratio of number of ShBRCA1-treated cells to ShLuc-treated cells, that is, ShBRCA1/ShLuc. Averages of the results of individual experiments are plotted. ( e ) BRCA1 mut/+ (CP10 and CP16) were transduced with shRNA directed at GAPDH (siGAPDH) or BRCA1 (siBRCA1). Three days post transfection, combinations of siGAPDH or siBRCA1-transduced BRCA1 mut/+ HMECs (CP10 and CP16) were co-plated with AR7 (a BRCA1 +/+ HMEC) and exposed to various doses of a PARP inhibitor. Averages of the results generated by these combinations were plotted. Error bars were calculated as the standard error propagation (SEP) in the ratios of each of the combinations in three independent experiments. Full size image When BRCA1 mut/+ and BRCA1 +/+ cells were compared for their sensitivity to olaparib, BRCA1 mut/+ cells were not found to be demonstrably sensitive ( Fig. 3b,c ). As a positive control, U20S cell line, made HR-DSBR incompetent by depleting BRCA1 (ShBRCA1 treated), was used along with control (ShLuc treated) cells. Once BRCA1 depleted, these cells proved to be highly sensitive to olaparib, while control cells were not ( Fig. 3d ). In addition, BRCA1 mut/+ HMEC viability was reduced by olaparib, again only after BRCA1 depletion (si BRCA1 , Fig. 3e ). Thus, despite the linkage of HR to BRCA1 breast cancer suppression and in keeping with results obtained in mouse ES cells [27] , these results, too, suggest that BRCA1 mut/+ cells are not defective for HR-dependent DSBR function. Stalled replication fork repair BRCA1 also protects the genome from DNA damage resulting at stalled replication forks [33] , [34] , [35] , [36] . It is rapidly attracted to these damage sites where it joins other proteins that are required for stalled fork repair (SFR). For example, BRCA1 is required for the generation of phospho-RPA32-coated single-stranded DNA (ssDNA), a pre-repair step needed for recruitment of ATRIP/ATR to activate the intra-S and G2/M checkpoints that support SFR [35] , [37] , [38] , [39] . In the absence of BRCA1, a stalled fork is more likely to be bypassed by translesional synthesis [35] , or, it may collapse into DSB, a hallmark of ‘replication stress’ and an established force in support of epithelial cancer development [40] , [41] . In the mammary epithelium, which undergoes normal periods of extreme proliferation (for example, during pubertal development and/or pregnancy), an accumulation of stalled forks, when not resolved, is likely to result in significant replication stress. Thus, we asked whether BRCA1 mut/+ cells are haploinsufficient in their ability to support SFR. Employing validated assays, we found that, by comparison with control cells, BRCA1 mut/+ fibroblasts and HMECs were defective in their SFR responses to replication-stalling agents like hydroxyurea (HU) and UV-C (ultraviolet radiation). We have shown previously that, in cells that were heavily depleted of BRCA1, recruitment of phospho-RPA32 (pRPA32) to chromatin was defective in response to UV [35] . This defect was also evident after treatment with HU ( Supplementary Fig. 4a ). When BRCA1 mut/+ cells were tested for their ability to recruit pRPA32 to chromatin after UV and/or HU treatment, a defect was detected in BRCA1 mut/+ cells ( Fig. 4a–c , and Supplementary Fig. 4a–d ). 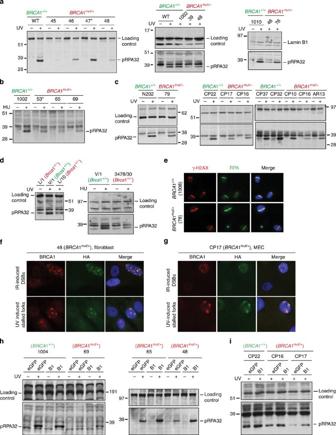Figure 4:BRCA1mut/+cells derived from human and mouse tissue are defective in the generation of phospho-RPA32-coated ssDNA. (a) Phospho-RPA32 (pRPA32) loading on chromatin is BRCA1 dependent. After UV-induced DNA damage,BRCA1mut/+fibroblasts exhibited reduced pRPA32 loading on ssDNA, compared withBRCA1+/+lines. Cells were irradiated with 30 J m−2of UV and harvested 3 h post damage. Chromatin extracts were prepared, and the relevant western blot was probed with an antibody to phosphorylated RPA32 (S4/S8). The replication status for each line was tested on the day of the experiment by BrdU uptake measurement, and only those lines that exhibited similar replication profiles were analysed. A subset of lines tested is shown here. Western blots for otherWTandBRCA1mutant lines are shown inSupplementary Fig. 4b. (b)BRCA1mut/+fibroblasts reveal reduced pRPA32 loading on ssDNA compared withBRCA1+/+lines, after HU exposure (10 mM for 3 h). An asterisk marks strains with the 185delAG mutation. (c)BRCA1mut/+HMECs reveal reduced pRPA32 loading on ssDNA, compared withBRCA1+/+HMECs after UV irradiation. (d) Mammary epithelial cells derived fromBrca1+/−(L/10 and 3478/30) and/orBrca1+/+(V/1) mice were analysed for pRPA32 levels on chromatin after UV- and HU-induced damage. (e)BRCA1mut/+cells efficiently recruit RPA32 to DSBs. RPA32 loading at laser-induced DSBs was equivalently efficient inBRCA1mut/+andBRCA1+/+lines. Cells were co-stained with anti- γ-H2AX to reflect the existence of DSBs. (f)BRCA1mut/+skin fibroblasts (48) and (g) mammary epithelial cells (CP17), each infected with a lentiviral vector expressing HA- tagged BRCA1, were either irradiated with 10 Gy IR (upper panel) or 30 J m−2of UV (lower panel). Cells were co-immunostained with Abs to BRCA1 and HA. (h,i) Phospho-RPA32 recruitment to ssDNA was analysed with a subset of primaryBRCA1mut/+andBRCA1+/+fibroblasts (h) and HMECs (i), infected with a lentiviral vector expressing either full-length WT BRCA1 (HA-tagged) or eGFP (control). Western blots were immunostained with Ab to phospho-RPA32. Figure 4: BRCA1 mut/+ cells derived from human and mouse tissue are defective in the generation of phospho-RPA32-coated ssDNA. ( a ) Phospho-RPA32 (pRPA32) loading on chromatin is BRCA1 dependent. After UV-induced DNA damage, BRCA1 mut/+ fibroblasts exhibited reduced pRPA32 loading on ssDNA, compared with BRCA1 +/+ lines. Cells were irradiated with 30 J m −2 of UV and harvested 3 h post damage. Chromatin extracts were prepared, and the relevant western blot was probed with an antibody to phosphorylated RPA32 (S4/S8). The replication status for each line was tested on the day of the experiment by BrdU uptake measurement, and only those lines that exhibited similar replication profiles were analysed. A subset of lines tested is shown here. Western blots for other WT and BRCA1 mutant lines are shown in Supplementary Fig. 4b . ( b ) BRCA1 mut/+ fibroblasts reveal reduced pRPA32 loading on ssDNA compared with BRCA1 +/+ lines, after HU exposure (10 mM for 3 h). An asterisk marks strains with the 185delAG mutation. ( c ) BRCA1 mut/+ HMECs reveal reduced pRPA32 loading on ssDNA, compared with BRCA1 +/+ HMECs after UV irradiation. ( d ) Mammary epithelial cells derived from Brca1 +/− (L/10 and 3478/30) and/or Brca1 +/+ (V/1) mice were analysed for pRPA32 levels on chromatin after UV- and HU-induced damage. ( e ) BRCA1 mut/+ cells efficiently recruit RPA32 to DSBs. RPA32 loading at laser-induced DSBs was equivalently efficient in BRCA1 mut/+ and BRCA1 +/+ lines. Cells were co-stained with anti- γ-H2AX to reflect the existence of DSBs. ( f ) BRCA1 mut/+ skin fibroblasts (48) and ( g ) mammary epithelial cells (CP17), each infected with a lentiviral vector expressing HA- tagged BRCA1, were either irradiated with 10 Gy IR (upper panel) or 30 J m −2 of UV (lower panel). Cells were co-immunostained with Abs to BRCA1 and HA. ( h , i ) Phospho-RPA32 recruitment to ssDNA was analysed with a subset of primary BRCA1 mut/+ and BRCA1 +/+ fibroblasts ( h ) and HMECs ( i ), infected with a lentiviral vector expressing either full-length WT BRCA1 (HA-tagged) or eGFP (control). Western blots were immunostained with Ab to phospho-RPA32. Full size image To test whether these abnormal RPA binding observations in BRCA1 mut/+ cells are specifically linked to BRCA1 haploinsufficiency, we asked whether ectopic wt BRCA1 expression in BRCA1 mut/+ cells corrects them. Infection by a lentiviral BRCA1 coding vector led to wt BRCA1 (HA-tagged) expression in primary BRCA1 mut/+ cells ( Fig. 4f,g ; Supplementary Fig. 5a ). This protein was recruited to DSBs and stalled forks in HMECs and fibroblasts like endogenous wt BRCA1 ( Fig. 4f,g ). Its expression suppressed the apparent, post-UV haploinsufficient defect in pRPA32 chromatin recruitment ( Fig. 4h,i , respectively). Thus, this defect is a valid representation of BRCA1 haploinsufficiency. To test the generality of SFR haploinsufficiency, we isolated MECs from Brca1 +/− and Brca1 +/+ mice. These cells were used to study the generation of phospho-RPA32-coated ssDNA after UV- and HU-induced stalled fork formation. In keeping with results obtained with BRCA1 heterozygous human cells, we observed reduced phospho-RPA32 coating of ssDNA in Brca1 +/− mouse cells compared with WT Brca1 +/+ cells ( Fig. 4d ). This underscores the generality of the finding that cells with one mutated allele for BRCA1 are haploinsufficient for pRPA32 loading on chromatin. pRPA32 loading on chromatin is dependent on the generation of ssDNA. Its generation after replication arrest is BRCA1 -dependent [35] . To detect the generation of ssDNA, a BrdU immunoassay [42] performed under non-denaturing conditions (HCl) was used. Here, using the same assay, we found that strain 39 ( BRCA1 mut/+ ) generated less ssDNA ( Supplementary Fig. 4e ,f) compared with strain 1002 ( BRCA1 +/+ ). This supports the hypothesis that BRCA1 mut/+ cells generate less ssDNA, which in turn results in less pRPA32 chromatin loading. Of note, 1075 (a human 185delAG /+ strain) failed to exhibit a defect in ssDNA generation. This suggests that the post UV generation of ssDNA was not affected in these cells and explains why we did not observe a defect in pRPA32 loading in them. Possibly, steps downstream of ssDNA generation and pRPA32 loading are defective in 185delAG strains (see for example, below). Finally, to test whether the inefficient loading of RPA at stalled forks in BRCA1 mut/+ cells is a reflection of innately reduced RPA activation after DNA damage, we assayed for RPA recruitment to DNA in response to UV laser-induced DSBs. As shown in Fig. 4e , RPA was equivalently recruited to these stripes in BRCA1 mut/+ and +/+ cells. This rules out the possibility of an innate defect in RPA activation after DNA damage. An inability to form pRPA32-coated ssDNA after DNA damage may result in relevant checkpoint defects [43] . Although we detected an incomplete reduction in pRPA32-coated chromatin after UV-induced DNA damage in BRCA1 mut/+ HMECs, there was no obvious S or G2 checkpoint defect. Thus, incomplete formation of pRPA32-coated ssDNA, in the conditions tested, was, nonetheless, sufficient to initiate a proper checkpoint response. Given that inefficient loading of pRPA32 on ssDNA is associated with an SFR defect, we asked whether BRCA1 mut/+ strains also experience an abnormally high frequency of collapsed forks compared with their WT counterparts ( BRCA1 +/+ ). Fork collapse can be captured by staining the cells with antibody to 53BP1 and/or γ- H2AX, which is routinely recruited to these damaged structures [35] , [44] . BRCA1 mut/+ cells, stained 18 h post UV with p-S1778 53BP1 and γ-H2AX Abs, revealed an increase in fork collapse by comparison with wt controls ( Fig. 5a,b ). This again implies that the efficiency of SFR is compromised in BRCA1 mut/+ cells, leading to higher fork collapse and incomplete resolution/repair of these structures. Thus, BRCA1 is haploinsufficient for the suppression of replication stress in primary HMECs and fibroblasts. 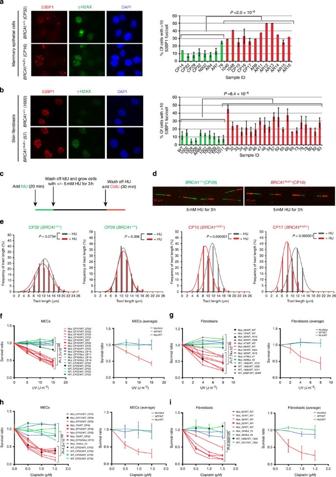Figure 5: The stalled fork repair pathway is defective inBRCA1mut/+cells. HeterozygousBRCA1mut/+cells reveal increased DNA break formation, after stalled fork-inducing DNA damage, show reduced replication fork stability, and are more sensitive than WTBRCA1+/+cells to stalled fork-inducing agents. After exposure to a stalled fork-inducing agent (UV and/or HU),BRCA1mut/+cells were prone to increased fork collapse compared withBRCA1+/+cells. (a) Skin fibroblasts, and (b) HMECs derived fromBRCA1mutation carriers (BRCA1mut/+) and wild typeBRCA1counterparts (BRCA1+/+), were irradiated with low dose UV (5 J m−2) and allowed to recover for 18 h. Cells were immunostained with Ab to 53BP1 and γ- H2AX (a marker for collapsed replication forks). The right (R) panel depicts the percentage of cells with ≥10 53BP1 foci per cell in HMECs and fibroblasts. Mean and s.d. of at least three experiments for each strain are shown (green: wtBRCA1+/+; red:BRCA1mut/+). (c) Schematic representation of DNA fibre experiment. (d) Representative tracts from DNA fibre experiments with HMECs (BRCA1+/+, CP29;BRCA1mut/+, CP10) treated with 5 mM HU for 3 h. Green and red tracts correspond to IdU and CldU incorporation, respectively. Red scale bar represents 10 μm length. (e) Distribution curves of IdU tract lengths in the presence and absence of HU (5 mM for 3 h) for bothBRCA1+/+(first two plots, CP32 and CP29) andBRCA1mut/+(last two plots, CP10 and CP17) cells. Red and Grey curves represent the presence and absence of HU in the culture medium, respectively. At least 200 tracts were scored for each distribution curve. (f,g) (Left panels) Combinations ofBRCA1mut/+andBRCA1+/+HMECs (f) and fibroblasts (g) were irradiated with different doses of UV. (Right) Average of data plotted on left. (h) Combinations ofBRCA1mut/+andBRCA1+/+HMECs and (i) fibroblasts were incubated with increasing concentrations of cisplatin for 15 h. Cells were allowed to recover for 6 days and then harvested for FACS analysis. Panels on the right show the averages of data plotted on the left. Figure 5: The stalled fork repair pathway is defective in BRCA1 mut/+ cells. Heterozygous BRCA1 mut/+ cells reveal increased DNA break formation, after stalled fork-inducing DNA damage, show reduced replication fork stability, and are more sensitive than WT BRCA1 +/+ cells to stalled fork-inducing agents. After exposure to a stalled fork-inducing agent (UV and/or HU), BRCA1 mut/+ cells were prone to increased fork collapse compared with BRCA1 +/+ cells. ( a ) Skin fibroblasts, and ( b ) HMECs derived from BRCA1 mutation carriers ( BRCA1 mut/+ ) and wild type BRCA1 counterparts ( BRCA1 +/+ ), were irradiated with low dose UV (5 J m −2 ) and allowed to recover for 18 h. Cells were immunostained with Ab to 53BP1 and γ- H2AX (a marker for collapsed replication forks). The right (R) panel depicts the percentage of cells with ≥10 53BP1 foci per cell in HMECs and fibroblasts. Mean and s.d. of at least three experiments for each strain are shown (green: wt BRCA1 +/+ ; red: BRCA1 mut/+ ). ( c ) Schematic representation of DNA fibre experiment. ( d ) Representative tracts from DNA fibre experiments with HMECs ( BRCA1 +/+ , CP29; BRCA1 mut/+ , CP10) treated with 5 mM HU for 3 h. Green and red tracts correspond to IdU and CldU incorporation, respectively. Red scale bar represents 10 μm length. ( e ) Distribution curves of IdU tract lengths in the presence and absence of HU (5 mM for 3 h) for both BRCA1 +/+ (first two plots, CP32 and CP29) and BRCA1 mut/+ (last two plots, CP10 and CP17) cells. Red and Grey curves represent the presence and absence of HU in the culture medium, respectively. At least 200 tracts were scored for each distribution curve. ( f , g ) (Left panels) Combinations of BRCA1 mut/+ and BRCA1 +/+ HMECs ( f ) and fibroblasts ( g ) were irradiated with different doses of UV. (Right) Average of data plotted on left. ( h ) Combinations of BRCA1 mut/+ and BRCA1 +/+ HMECs and ( i ) fibroblasts were incubated with increasing concentrations of cisplatin for 15 h. Cells were allowed to recover for 6 days and then harvested for FACS analysis. Panels on the right show the averages of data plotted on the left. Full size image Of note, 185delAG -bearing strains (that is, 26, 47, 53, 57, AR19L) exhibited near normal loading of pRPA32 onto chromatin (marked with asterisk in Fig. 4a and Supplementary Fig. 4b ), but more abundant 53BP1 foci by comparison with control cells ( Fig. 5b ). Others have shown that the 185delAG allele expresses a modestly truncated BRCA1 protein, translation of which is initiated immediately downstream of the mutation near the 5′ end of the gene [45] . Thus, one might hypothesize that 185delAG is a hypomorph, capable of supporting some but not all BRCA1 SFR support functions. To better understand the fate of collapsed forks in BRCA1 mut/+ cells, we carried out DNA fibre analysis. We wished to assess two phenotypes: (1) the stability of nascent replication tracts after fork stalling and (2) the efficiency of replication restart. Cells were pulse labelled with IdU for 20 min followed by treatment with or without 5 mM HU for 3 h. After washing off HU, cells were incubated in the presence of CldU for 30 min ( Fig. 5c ). This protocol allows the analysis of the fate of nascent replication tracts (synthesized before HU addition) during replication stalling, as well as replication fork restart after a replication block is eliminated ( Fig. 5c ). DNA fibre assays have been used previously with Brca1 −/− mouse ES cells to show that BRCA1 is required to suppress degradation of nascent strands after replication stalling induced by HU treatment [36] . In that study, replication restart was not affected by the absence of BRCA1. In keeping with these results, we find that, in the presence of HU, BRCA1 mut/+ cells exhibited increased degradation of the nascent strand (shorter green tracts) at stalled forks compared with the BRCA1 +/+ cells ( Fig. 5d,e ; Supplementary Fig. 5c ). As shown in Fig. 5e , the distribution of nascent DNA tract lengths (green tracts, Fig. 5d ) for BRCA1 +/+ MECs (CP32 and CP29) was not different between HU-treated and -untreated samples (red and grey curves, respectively). However, the red curves shifted towards shorter lengths (increased degradation) after treatment with HU in BRCA1 mut/+ cells (CP10 and CP17). By contrast, no significant difference in the ability of BRCA1 mut/+ cells to restart replication was detected after replication stress had abated ( Fig. 5c–e ; Supplementary Fig. 5c ). These results further support our conclusion that the stability of stalled forks is compromised in BRCA1 heterozygous ( BRCA1 mut/+ ) cells. To assess further the conclusion that inefficient SFR in BRCA1 mut/+ cells results in increased DNA breaks, we employed comet assays. In UV-treated cells there was a greater increase in DNA breaks in BRCA1 mut/+ when compared with BRCA1 +/+ cells ( Supplementary Fig. 5d,e ). This result reaffirms the finding that, faced with replication stalling, BRCA1 heterozygous primary cells exhibited signs of replication stress, unlike BRCA1 +/+ cells. Roles of BRCA1 -associated proteins in SFR in BRCA1 mut/+ cells A stalled fork serves as a scaffold to recruit and concentrate proteins that play critical role/s in stabilizing, processing, repairing and restarting a stalled fork. This is essential to prevent the risk of its collapse into a DSB, a prime contributor to genomic instability. We tested a subset of the proteins that are known to be recruited to a stalled fork, with an eye towards those that interact and/or function together with BRCA1 to carry out SFR. Specifically, we asked whether recruitment of Rad51, a BRCA1 partner in HR-based DSBR [46] , [47] and a protein known to play an HR-independent repair role at stalled forks [48] , is affected in BRCA1 mut/+ cells. We found that Rad51 recruitment to UV-induced stalled forks was reduced in BRCA1 mut/+ compared with BRCA1 +/+ cells ( Supplementary Fig. 6b ). This was not surprising, given that Rad51 is recruited to RPA-coated ssDNA, the generation of which is compromised in BRCA1 mut/+ cells. We also found that the same BRCA1 mut/+ strains that revealed efficient Rad51 recruitment to DSBs ( Fig. 2e,f ) were defective in recruiting Rad51 to stalled forks. This implies that the role of Rad51 at a stalled fork is different from that at a DSB and further confirms the observations made by other groups who found that Rad51 helps restart stalled forks in an HR-independent manner [36] , [48] , [49] . In addition, Scully et al. [50] detected significant differences between the mechanism of repair at a non replication fork-associated DSB and at a stalled fork-induced break. We next assayed the efficiency of CtIP recruitment to UV-induced stalled forks. CtIP is an established BRCA1 partner [51] and plays an important role in replication restart after stalled fork formation [52] , [53] . We found previously that BRCA1 is required for the recruitment of CtIP to UV-induced stalled forks [35] . In light of this evidence, we asked whether CtIP recruitment is compromised in BRCA1 mut/+ cells. Just as for Rad51, BRCA1 mut/+ cells exhibited reduced CtIP recruitment to sites of UV-induced fork stalling ( Supplementary Fig. 6a ). It is unclear whether this defect in CtIP recruitment to stalled forks is a direct result of a reduced BRCA1 protein level or reduced pRPA32-coated ssDNA. Nonetheless, these data further confirm that BRCA1 mut/+ cells are defective in SFR. Finally, we addressed the fate of Mre11 at stalled forks in BRCA1 mut/+ and BRCA1 +/+ cells. Mre11 is a BRCA1-associated nuclease that has been implicated in helping restart collapsed and stalled replication forks via resection and initiation of repair at these sites [49] , [54] , [55] . Given that BRCA1 mut/+ cells exhibit reduced ssDNA generation, defective pRPA32 loading on chromatin and collapsed forks, we asked whether Mre11 recruitment mirrors this phenotype. The data revealed increased Mre11 recruitment to the sites of UV-induced stalled forks in BRCA1 mut/+ cells compared with BRCA1 +/+ cells ( Supplementary Fig. 6c ). Given that Mre11 is a nuclease that is recruited to DSBs, it seems reasonable to propose that increased fork collapse in BRCA1 mut/+ cells results in DSBs, that, in turn, recruit Mre11. Thus, in lieu of possibilities discussed above, increased Mre11 recruitment to UV-induced stalled forks in BRCA1 mut/+ cells may be yet another indicator of the reduced stability of stalled forks in BRCA1 mut/+ cells. Cell sensitivity to different DNA damage inducing agents In an effort to validate the observation that primary BRCA1 mut/+ cells are defective for SFR and suppression of replication stress, the relative sensitivity of these primary cells to stalled fork-inducing agents, like UV and cisplatin [56] , was tested in differentially coloured, co-cultured cells. In multiple comparisons of primary BRCA1 mut/+ and BRCA1 +/+ fibroblasts and HMECs, the heterozygotes were significantly more sensitive than the wt cells to UV ( Fig. 5e,f ) and cisplatin ( Fig. 5g,h ). HR-DSBR in BRCA1 mut/+ cells undergoing replication stress The discordance between multiple intact and one defective BRCA1-associated functions in numerous, primary heterozygous cell strains suggests that BRCA1 mut/+ cells can preferentially direct their limited stores of intact BRCA1 protein to checkpoint activation, HR-DSBR, centrosome, SLUG control and spindle pole function, and less effectively to SFR. Alternatively, less BRCA1 protein is required for the former functions than the latter one. In either case, we asked whether, when these cells encounter sufficient replication stress, BRCA1 becomes preferentially dedicated to SFR and, in doing so, the pool of BRCA1 available for otherwise intact functions is reduced. If it falls sufficiently, do BRCA1 mut/+ cells now become multiply haploinsufficient, that is, for other known BRCA1 functions that were formerly intact in these cells. To address this possibility, we pre-exposed cells to increasing doses of UV and then assayed them for other BRCA1 functions (other than SFR). To assay for HR, the UV-treated cells were irradiated with IR and analysed for recruitment of Rad51 to DSBs ( Fig. 6a ). To assay for spindle formation and centrosome maintenance, we allowed the cells to recover for one and/or two full cycles of cell division and then analysed the cells for spindles as well as centrosomes. 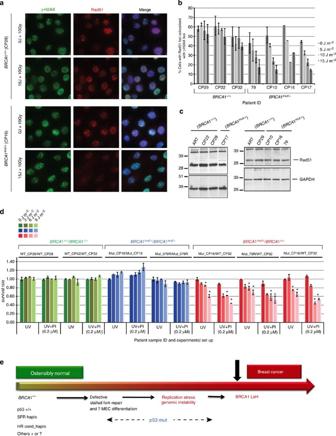Figure 6: Evidence of conditional haploinsufficiency for DSBR inBRCA1mut/+HMECs after pre-exposure to a stalled fork- inducing agent. (a) Recruitment of Rad51 to IR-induced DSBs is reduced in heterozygousBRCA1mut/+, and not in WTBRCA1+/+HMECs, when pre-exposed to stalled fork-inducing damage. HMECs derived from aBRCA1mutation carrier (CP16,BRCA1mut/+) and a wt counterpart (CP29,BRCA1+/+) were irradiated with different doses of UV (5, 10 or 15 J m−2) and allowed to recover for 1 h. Cells were then irradiated with IR (10 Gy) and fixed 4 h post IR. Fixed cells were coimmunostained with Abs to γ-H2AX and Rad51. Additional wt and heterozygous strains were also assayed (in panelb). (b) AdditionalBRCA1+/+andBRCA1mut/+strains were analysed as described in (a). A graph depicting the fraction of cells in each additional HMEC strain that contains Rad51 foci after exposure to increasing doses of UV followed by 10 Gy dose of IR was plotted. The mean results and s.d. of data from at least three experiments are shown for each line. (c) Rad51 expression inBRCA1mut/+andBRCA1+/+HMEC lines. Whole-cell extracts from variousBRCA1mut/+andBRCA1+/+strains were analysed by western blot. GAPDH was used as a loading control in these blots. (d) Combinations ofBRCA1mut/+andBRCA1+/+HMECs (green:BRCA1+/+/BRCA1+/+, blue:BRCA1mut/+/BRCA1mut/+and red:BRCA1mut/+/BRCA1+/+) were irradiated with different doses of UV (0, 3, 6 and 9 J m−2), allowed to recover for 1 h, and then treated with either 0.2 μM PARP inhibitor (PI=olaparib; UV+PI) or DMSO as control (UV). Cells were grown for five more days before harvesting for FACS analysis. Data are plotted for the three, different cell combinations, and the error bars were calculated as the standard error propagation (SEP) in the ratios of each of the combinations in three, independent experiments. Data marked with an asterisk (*) reveal statistically significant differences (P-value<0.05) between UV and UV+PI sets. (e) One Possible Model ofBRCA1mutation- driven tumorigenesis. This model speculates that certain abnormal developments might occur during the extended period between full mammary development and the appearance of aBRCA1breast cancer. Figure 6: Evidence of conditional haploinsufficiency for DSBR in BRCA1 mut/+ HMECs after pre-exposure to a stalled fork- inducing agent. ( a ) Recruitment of Rad51 to IR-induced DSBs is reduced in heterozygous BRCA1 mut/+ , and not in WT BRCA1 +/+ HMECs, when pre-exposed to stalled fork-inducing damage. HMECs derived from a BRCA1 mutation carrier (CP16, BRCA1 mut/+ ) and a wt counterpart (CP29, BRCA1 +/+ ) were irradiated with different doses of UV (5, 10 or 15 J m −2 ) and allowed to recover for 1 h. Cells were then irradiated with IR (10 Gy) and fixed 4 h post IR. Fixed cells were coimmunostained with Abs to γ-H2AX and Rad51. Additional wt and heterozygous strains were also assayed (in panel b ). ( b ) Additional BRCA1 +/+ and BRCA1 mut/+ strains were analysed as described in ( a ). A graph depicting the fraction of cells in each additional HMEC strain that contains Rad51 foci after exposure to increasing doses of UV followed by 10 Gy dose of IR was plotted. The mean results and s.d. of data from at least three experiments are shown for each line. ( c ) Rad51 expression in BRCA1 mut/+ and BRCA1 +/+ HMEC lines. Whole-cell extracts from various BRCA1 mut/+ and BRCA1 +/+ strains were analysed by western blot. GAPDH was used as a loading control in these blots. ( d ) Combinations of BRCA1 mut/+ and BRCA1 +/+ HMECs (green: BRCA1 +/+ / BRCA1 +/+ , blue: BRCA1 mut/+ / BRCA1 mut/+ and red: BRCA1 mut/+ / BRCA1 +/+ ) were irradiated with different doses of UV (0, 3, 6 and 9 J m −2 ), allowed to recover for 1 h, and then treated with either 0.2 μM PARP inhibitor (PI=olaparib; UV+PI) or DMSO as control (UV). Cells were grown for five more days before harvesting for FACS analysis. Data are plotted for the three, different cell combinations, and the error bars were calculated as the standard error propagation (SEP) in the ratios of each of the combinations in three, independent experiments. Data marked with an asterisk (*) reveal statistically significant differences ( P -value<0.05) between UV and UV+PI sets. ( e ) One Possible Model of BRCA1 mutation- driven tumorigenesis. This model speculates that certain abnormal developments might occur during the extended period between full mammary development and the appearance of a BRCA1 breast cancer. Full size image As shown in Fig. 2e,f , multiple BRCA1 mut/+ and BRCA1 +/+ cell strains recruited Rad51 to IR-induced DSBs with equal efficiency in the absence of UV pre-treatment. However, the ability of BRCA1 mut/+ cells to recruit Rad51 to DSBs became increasingly defective after exposure to increasing doses of UV ( Fig. 6a,b ). No such effect was detected in BRCA1 +/+ cells. We asked whether changes in BRCA1 protein levels in the UV pre-treated heterozygotes could account for reduced Rad51 recruitment, but no obvious alterations were observed ( Supplementary Fig. 4e ). This result, along with the observation that Rad51 protein levels in BRCA1 mut/+ and BRCA1 +/+ were also similar ( Fig. 6c ), suggests that a defect in Rad51 recruitment to DSBs, in UV- pretreated BRCA1 mut/+ cells, is a result of a defect in the ability of a limited pool of BRCA1 protein to respond to DSBs by driving the HR-DSBR process. To assess further the apparent emergence of ‘conditional haploinsufficiency’ for HR-DSBR in the presence of replication stress, we used the FACS-based assay described earlier to determine the survival efficiency of BRCA1 mut/+ cells in the presence of olaparib. The question here was whether pre-exposure of cells to stalled fork-inducing damage (for example, UV) compromises the ability of these cells to carry out DSBR. If so, the BRCA1 mut/+ cells should become olaparib-sensitive. Evidence presented in Fig. 6d showed this to be the case. Exposure of BRCA1 mut/+ cells to increasing doses of UV before adding olaparib rendered them acutely sensitive to a relatively low concentration of olaparib ( Fig. 6d ). Centrosome number and spindle formation in the same cell strains were not altered under these conditions (data not shown). This implies that, at the very least, there is conditional haploinsufficiency [57] for HR-DSBR in BRCA1 mut/+ cells facing sufficient replication stress. Multiple primary fibroblast and HMECs derived from non-tumour tissue of BRCA1 mutation carriers reveal, for the first time, the existence of BRCA1 haploinsufficiency for one of its established, genome integrity maintenance functions, that is, its ability to support SFR and to prevent replication stress. By contrast, no such defect was detected among several other such functions. Conceivably, haploinsufficiency for some of these apparently unaffected BRCA1 functions occurs but takes considerably longer to develop during the life of a BRCA1 mut/+ individual than did the defect in SFR. In addition, the quantity of BRCA1 needed to sustain at least some of its other functions may be significantly less than that required for this activity. Furthermore, in keeping with a model first proposed by Bartek et al. [57] , the data presented here also reveal a possible hierarchy of DNA repair functions in BRCA1 mut/+ cells, wherein a defect in SFR, if not resolved, can trigger an otherwise undetectable defect in HR-DSBR following enhanced replication stalling. In effect, representative primary BRCA1 mut/+ HMECs and fibroblasts exhibited a state of innate haploinsufficiency for SFR and ‘conditional’ haploinsufficiency for HR-DSBR. Thus, in keeping with the model of Bartek et al. [57] , we hypothesize that, when the amplitude of replication stalling rises above a threshold level in cells that are already deprived of a full complement of intact BRCA1, the available BRCA1 pool is dedicated first to preventing and repairing collapsed forks. This leaves even less BRCA1 available to form complexes that are required for the execution of HR at DSB that are not associated with fork collapse. The latter effect can be hypothesized to give rise to the de novo development of an HR defect. This prediction was borne out experimentally. Why replication stress did not affect any other BRCA1 genome integrity maintenance function, other than HR-DSBR, is unknown. One possible explanation is that BRCA1 appears to execute each of these unaffected functions as a member of a large, multi-subunit complex(es) [4] , [15] , [21] , [58] , [59] . Conceivably, these complexes are sufficiently stable, well-compartmentalized and function efficiently enough before the onset of replication stalling that they are not disadvantaged by such an event. Given the strong contributory history of inadequate SFR to epithelial cancer development and the fact that it is, thus far, the only apparent haploinsufficient BRCA1 DNA repair abnormality, we speculate that SFR haploinsufficiency serves as an early and persistent contributor to the long process that gives rise to BRCA1 breast cancer ( Fig. 6e ). The fact that, when exposed to sufficient levels of replication stress, conditional BRCA1 HR-DSBR haploinsufficiency emerged in BRCA1 heterozygous cells suggests that this defect might join SFR haploinsufficiency as a BRCA1 breast cancer co-contributor in mammary epithelial progenitor cells that are experiencing sufficient ongoing replication stress. This would befit its widely accepted role as a major BRCA1 breast cancer risk factor. Assuming that other BRCA1 functions remain to be discovered, it is conceivable that one or more of them, too, is haploinsufficient in the cells we have analysed. Thus, the current picture, while new, may be incomplete. BRCA1 haploinsufficiency for SFR was also apparent in Brca1 +/− mouse MECs. Given that Brca1 +/− mice are not tumour prone [60] , this suggests that haploinsufficiency for SFR in mMECs is not sufficient to drive tumorigenesis, especially given the short life span of mice. Furthermore, despite the tissue specificity (breast and ovary) of BRCA1 mutant cancer, a haploinsufficient phenotype was not limited to mammary epithelial cells. Similar defects were also displayed by BRCA1 mut/+ fibroblasts, thereby supporting the notion that multiple factors combine to generate the tissue specificity of BRCA1 -mutant cancer. Indeed, while drafting this manuscript, a new haploinsufficient role for BRCA1 was reported [61] . The authors showed that transcription of the CYP1A gene, which encodes an estrogen-metabolizing enzyme, is upregulated in BRCA1 heterozygous cells [61] . In addition, Savage et al. [61] showed that these oestrogen metabolites result in increased DNA damage in BRCA1 heterozygous cells. In light of the existence of defective SFR in BRCA1 heterozygous cells, it is reasonable to predict that such a defect would be a key avenue through which haploinsufficiency for oestrogen metabolite detoxification could result in DNA damage. Even if SFR haploinsufficiency was not the only DNA repair defect in BRCA1 heterozygous HMECs, the high potential for it to give rise to chronic replication stress may well be clinically significant. This is because chronic replication stress is an established and common force in human epithelial cancer formation [40] , [41] , [62] , [63] . Moreover, others have observed defects in differentiation in populations of primary BRCA1 mut/+ HMECs [8] , [9] , [10] , [11] . As yet undefined BRCA1 functional abnormalities underlie this set of phenotypes and could, when deciphered, enlarge the results described here. The extent to which SFR and, possibly, conditional HR-DSBR haploinsufficiency contribute to them is unknown but worthy of investigation. DNA damage is known to perturb the differentiation of certain cell types [64] . Recently, Winqvist et al. [65] reported the existence of haploinsufficiency for replication stress responsiveness in EBV-immortalized B lymphocytes and primary T cells derived from PALB2 heterozygotes. Their ability to perform HR was not analysed. These data obtained from cells with a single PALB2 mutant genotype represent an example of haploinsufficiency for a known BRCA1- and BRCA2- interacting protein that is also a breast cancer suppressor. Thus, those results and evidence reported here imply that haploinsufficiency in replication stress suppression is a feature of ostensibly normal mammary epithelial cells of two, different sets of mutation carriers. In this regard, evidence of BRCA1 haploinsufficiency was sought by Buchholz et al. [66] in BRCA1 heterozygous fibroblasts and lymphocytes, and by Konishi et al. [28] in a human HMEC line where a BRCA1 mutation (185delAG) was introduced into one allele by gene targeting. Buchholz et al. [66] observed increased sensitivity of BRCA1 heterozygous fibroblasts to ionizing radiation (IR) and increased chromatid breaks in lymphocytes after IR. Given the pleiotropic effect of IR on DNA (for example, strand breaks, fork stalling, base damage, DNA-adducts [67] , [68] , [69] ), one cannot rule out that the sensitivity to IR is a result of contribution of multiple forms of DNA damage and not just a response to DSB formation. Similarly, in Konishi et al. [28] it was suggested that the targeted heterozygous clones were defective in HR-DSBR. Although increased sensitivity of these clones to IR and a reduced HR-DSBR signal in HR reporter-containing cells were detected, they, like we, failed to observe any sensitivity of their BRCA1 mut/+ cells to PARP inhibition, raising a question regarding the existence of an HR defect. Given that the test cells were reported to be slow to proliferate, this could have contributed towards apparent HR deficiency. The possibility that persistent replication stress is a tumour-promoting force in BRCA1 mut/+ mammary epithelial cells offers, a hypothetical, mechanism-based route to BRCA1 breast cancer prevention. If specific subsets of BRCA1 mut/+ HMECs normally advance beyond the manifestation of an SFR defect to develop additional BRCA1 functional deficiencies accompanied by a much higher risk of tumorigenicity, their selective elimination might suppress subsequent BRCA1 breast cancer development. Isolation and culture of human MECs and fibroblasts from tissue biopsies Tissue samples were briefly washed in PBS and then minced and digested overnight at 37 °C in medium containing 1 mg ml −1 of collagenase type III (Roche). For digestion, MEGM medium (Lonza) was used for breast tissue, and Dulbecco’s modified Eagle’s Medium (DMEM) with 5% fetal bovine serum (FBS) for skin tissue. The digested tissue was pelleted and fibroblasts were cultured in DMEM supplemented with 15% FBS (Gibco), 1% Pen/Strep (Gibco) and 1% Glutamine (Gibco), and HMECs were grown in MEGM medium supplemented with 1% Pen/Strep. Isolation and culture of mouse MECs from mouse mammary tissue Primary mouse MEC cultures were generated from the 4th and 5th pairs of mammary fat pads using a sterile technique. The tissue was digested overnight at 37 °C in serum-free Leibovitz-15 medium containing 3 mg ml −1 of collagenase A (Sigma). Digestion was stopped by adding 1 × volume of 10% serum containing DMEM. The pelleted cells and organoids were plated and cultivated in DMEM/F12 50:50 medium supplemented with 10% FCS, 50 units ml −1 penicillin, 50 μg ml −1 streptomycin (Life Technologies), 5 μg ml −1 recombinant human insulin (Sigma), 5 ng ml −1 recombinant human EGF (Sigma) and 5 ng ml −1 cholera toxin (Calbiochem). Mouse model and genotyping The mouse Brca1 null allele used in this study was generated by crossing mice harbouring the BRCA1F5-13 conditional allele (kindly provided by Dr Jos Jonker’s group) [60] with Meox2-Cre deleter mice purchased from Jackson Labs (Bar Harbor, ME—Stock #003755). Mouse genotyping was performed on genomic DNA extracted from mouse-tail snips using standard procedures [60] . Genotyping for Cre-generated Brca1 null allele was carried out with primers GenoB1-A (5′-AGGTACCAGTTATGAGTTAGTCGTGTGCCTGAGTCA-3′) and GenoB1-D (5′-GGCTACCTATAACTACTCTCTAACAACGAAGTGCAA-3′), which yielded a 654-bp fragment. The wt brca1 allele was genotyped using primers GenoB1-A and GenoB1-B (5′-GCTGAGATTAAAGTGCAGGCCACCACACTCAGTGAT-3′), which yielded a PCR product of 495 bp for the wt allele and 624 bp for the floxed allele. PCR amplification conditions used were as described previously [60] . Primers Meox2Cre1 (5′-CCTGAAAGCAGTTCTCTGGGACCACCTTCTTTTGGCTTC-3′) and Meox2Cre2 (5′-CTTCTTCTTGGGTCCTCCCAGATCCTCCTCAGAAATCAGC-3′) were used to verify the presence of Meox2 Cre allele. Amplified fragment was 423 bp. Transfection, infection and selection For siRNA experiments, cells were grown in six-well plates and transfected with 100 pmoles of siRNA with RNAiMAX (Invitrogen) according to the manufacturer’s protocol. Where relevant, experiments were initiated 48 h after transfection. All siRNA oligonucleotides were purchased from Thermo Scientific. siRNA oligonucleotides used were siBRCA1 (On Target Plus BRCA1, catalog number CTM-41735) and siGAPDH (On Target Plus GAPDH, catalog number D-001830-01-20). For shRNA experiments, shRNA encoding lentiviruses were generated using 293FT-packaging cells in the presence of lipofectamine (Invitrogen). Cells infected with puroR-encoding lentiviruses were selected transiently using 2.5 μg ml −1 puromycin (Santa Cruz). ShBRCA1 and shLuc were acquired from The RNAi Consortium (TRC). The target sequence for shBRCA1 was 5′-AGAATCCTAGAGATACTGAA-3′. For BRCA1 reconstitution experiments, lentiviral packaging plasmids, VSVG and PSPAX, were used to package BRCA1 and/or eGFP plasmids in 293FT cells using lipofectamine (Invitrogen). Cells were infected with the lentivirus and selected using 6 μg ml −1 of Blasticidin (Invitrogen). For colour-coding experiments, hTERT and GFPhTERT containing retroviruses were prepared by packaging the plasmids pMIG-hTERT and pBABE-hygro-hTERT with the retrovirus packaging plasmids, pMD-MLV and pMD-G, in 293FT cells. hTERT-infected cells were selected with hygromycin B (Roche) (50 μg ml −1 ). Immnoblotting and antibodies Whole-cell extracts were prepared by lysing cells in NETN300 lysis buffer (300 mM NaCl, 20 mM Tris–HCl buffer pH7.8, 0.5% NP-40, 1 mM EDTA) for 1 h at 4 °C. Nuclear extracts were prepared by pre-extracting the cytoplasmic protein fraction by incubating the cells in pre-extraction buffer, that is, PEB (0.5% Triton -X-100, 20 mM HEPES pH 7.0, 100 mM NaCl, 3 mM MgCl 2 and 300 mM Sucrose). Incubation was carried out at 4 °C for 20 min. Cells were pelleted, washed once in PEB, and lysed in NETN 400 lysis buffer (400 mM NaCl, 20 mM Tris-HCl buffer pH7.8, 0.5% NP-40, 1 mM EDTA) for 45 min at 4 °C. All lysis buffers were supplemented with 1 × protease inhibitor (Roche) and Halt Phosphatase inhibitor (Thermo Scientific). Chromatin extracts were prepared as described previously [43] . Immunoprecipitation for HA- tagged BRCA1 was carried out by incubating whole-cell extracts with an HA antibody (Covance) for 2 h, followed by 1 h incubation with Protein A beads (GE healthcare) at 4°C. The beads were washed in NETN 150 buffer (150 mM NaCl, 20 mM Tris–HCl buffer pH7.8, 0.5% NP-40, 1 mM EDTA). Antibodies used for western blotting were phospho-RPA32 (Bethyl Labs, A300-245A; 1:2,000), BRCA1 (SD118; 1:1,000), GAPDH (Santa Cruz, SC-25778; 1:4,000), pS53BP1-S25 (Novus Biologicals, NB100-1803; 1:5,000), Rad51 (Santa Cruz, SC-8349; 1:600), Slug (Cell Signaling, C19G7; 1:3,000), Vinculin (Santa Cruz, SC-55465; 1:1,000), BRCA1 (MS110; 1:1,000) and HA (Covance, MMS-101P; 1:4,000). Uncropped western blots for Figs 1,4,6, and Supplementary Figs 2–5 are shown in Supplementary Fig. 7. Immunofluorescence and antibodies Cells on coverslips were fixed with 4% paraformaldehyde/2% Sucrose for 15 min, and triton extracted (0.5% Triton X-100 in PBS) for 4 min. Cells were blocked with 5%BSA/PBST and then incubated with respective antibodies for 30 min at 37 °C followed by incubation with secondary antibodies (FITC or Rhodamine) for 30 min at 37 °C. Primary antibodies used in immunofluorescence studies were BRCA1 (Upstate; 1:500), phospho-53BP1(S1778) (Cell Signaling, 2675S; 1:200), RPA (Cal Biochem, NA13; 1:100), 53BP1 (Bethyl Labs, A300-272A; 1:2,000), Rad51(Santa Cruz, SC-8349; 1:150), Mre11 (Genetex, GTX70212 1:200), CtIP (generous gift from Dr. Richard Baer), HA (Covance, MMS-101P; 1:500) and γ-H2AX (Millipore, 05-636; 1:5,000). For TPX2 (Bethyl Labs, A300-429A; 1:400) and γ-tubulin (Sigma- Aldrich, T6557; 1:1,000) staining, the cells were pre-fixed with acetone:methanol (3:7) at −20 °C for 10 min, followed by triton extraction (0.2% triton-X-100 in 20 mM HEPES, pH 7.4, 50 mM NaCl, 3 mM MgCl2, 300 mM Sucrose) at room temperature. Primary and secondary antibody staining was carried out as described above. Cell treatments For analysis of phospho-RPA32 loading on chromatin, cells were treated with stalled fork inducing agents like HU (Sigma) and/or UV. Cells were incubated in HU (10 mM)-containing medium for 4 h before harvesting for further analysis. For UV treatment, cells were irradiated with 30 J m −2 UV with a 254 nm UV-C lamp (UVP Inc., Upland, CA) and harvested 4 h post UV. UV-irradiation through a micropore membrane was performed as described previously [43] . For colour- coded FACS-based cell survival assays, the Parp inhibitor, olaparib (Selleck), was added at final concentrations of 0.2, 0.4 and 0.6 μM for 6 days. cisplatin (Novaplus) was added at final concentrations of 0.5, 1.0 and 1.5 μM for 24 h. Medium was replaced, and the cells were allowed to grow for five more days. The doses of UV used were 5, 10 and 15 J m −2 , and cells were allowed to recover for 6 days before they were harvested for FACS analysis. Laser-induced DNA breaks were generated as described in Greenberg et al. [4] DNA fibre assay DNA fibres were prepared and analysed as described previously [48] , [49] with a few modifications. In brief, cells were labelled with 25 μM IdU for 20 min, washed two times and incubated in presence of 5 mM HU for 3 h. This was followed by incubation with 250 μM CldU for 30 min. Labelled cells were harvested, mixed 1:5 with unlabelled cells, lysed and spread on slides to obtain single-DNA tracts. After fixation, denaturation and blocking, the DNA tracts were stained with rat anti-CldU (Abcam, ab6326), followed by staining with a secondary antibody Alexa fluor 555 goat anti-rat overnight at 4 °C. DNA tracts were then stained with mouse anti- IdU (BD Biosciences, 555627) followed by a secondary antibody Alexa- 488 goat anti mouse. ImageJ software was used for determining the tract lengths based on scale bar generated during microscopy. Detection of ssDNA (BrdU ssDNA Assay) BrdU ssDNA assay was performed as described previously [42] . In brief, cells on coverslips were cultured with 30 mM BrdU for 20 h, and then released in BrdU-free medium for 16 h. Cells were stained as described previously [42] . Sequencing and hME Cells lines were sequenced to confirm their mutations via direct sequencing or by the hME sequencing method. Genomic DNA was prepared from Blood and a DNeasy kit (Qiagen), and a mutation locus-specific PCR reaction was carried out to amplify the region of interest. For direct sequencing, the amplified PCR products were purified using a Qiagen PCR purification kit and were sent for sequencing. For hME analysis, a locus-specific primer extension reaction of the PCR amplified region was carried out in the presence of a mixture of di-deoxy and deoxy NTPs. Allele-specific extension products were analysed by mass spectrometry to determine the specific sequence. More details of the protocol are available at the following link: http://cancer-seqbase.uchicago.edu/documents/AssayDesign3.1Guide.pdf Comet assay and analysis For detection of DNA breaks, alkaline comet assays were performed using the Single-Cell Gel Electrophoresis Assay kit (Trevigen) according to the manufacturer’s instructions. The quantification of tail DNA was carried out using CellProfiler software. Flow cytometry, checkpoints and colour-coding-based cell survival FACS assay For cell cycle analysis, cells were pulse-labelled with 10 μM BrdU for 30 min (for HMECs) and 1.5 h (for fibroblasts) in respective culture media. Single-cell suspensions were fixed in 70% ice-cold ethanol. Cells were incubated with an anti-BrdU FITC conjugate antibody (Becton Dickinson, 1:10 dilution made in Blocking solution from Thermo Scientific) at room temperature in the dark for 45 min. Finally, the cells were resuspended in propidium iodide and RNAse staining buffer (Becton and Dickinson) and analysed using a Becton Dickinson FACS (Mountain View, CA). For checkpoint assays, cells were irradiated with UV and/or IR and allowed to recover for 2 h. For S-phase checkpoint analysis, cells were incubated with BrdU, as described above, before harvesting and fixing for FACS analysis. For G2 checkpoint, fixed cells were incubated with an Alexa Fluor anti-phospho-histone H3 (Ser10) antibody diluted in 2% BSA/PBS at room temperature in the dark for 2 h. Cells were washed and resuspended in propidium iodide and RNAse-containing staining buffer. For colour-coded FACS-based assays, GFP-positive and -negative cells were mixed in equal numbers (8,000 cells per strain) and plated in 6 cm 2 plates. After drug and/or UV treatment, cells were allowed to recover for 6 days before being harvested for FACS analysis. Satellite RNA q-RT-PCR Cells grown in 6 cm 2 plates were collected, RNA was prepared using an RNeasy Plus Mini Kit (Qiagen), followed by cDNA preparation. q-RT-PCR was carried out with primers for SatA, SatIII, mcbox and β-Actin. More details and primer sequences are described in Zhu et al. [18] How to cite this article : Pathania, S. et al. BRCA1 haploinsufficiency for replication stress suppression in primary cells. Nat. Commun. 5:5496 doi: 10.1038/ncomms6496 (2014).